Cooperative material transport during the early stage of sintering The complex transport processes contributing to sintering are not yet fully understood, partially because in-situ observations of sintering in three dimensions (3D) are very difficult. Here we report a novel experiment in which monocrystalline copper spheres are first marked with microscopic boreholes drilled using a focused ion beam, after which high-resolution synchrotron X-ray tomography is carried out to measure translational, rolling and intrinsic rotation movements of some hundred spheres during sintering. Unlike in 1D and 2D systems, we show that, in 3D, intrinsic rotations are more pronounced than angular rolling rearrangements of the particle centres and become the dominant mechanism of particle movement. We conclude that in addition to the well-known neck growth and centre approach mechanisms, grain boundary sliding caused by the different crystallographic orientations of the individual spheres occurs. Sintering transforms a disperse state of matter into a solid body with higher density. Prominent examples in nature are the formation of ice glaciers from snow, or sandstone from sand particles. In industrial applications, sintering is the basis for the production of ceramics and a great variety of metallic and composite materials [1] , [2] , [3] . Depending on the technology and type of material chosen, the initial powder particle size may range from several hundreds of μm down to about 10 nm. At temperatures below the melting point, solid-state diffusion allows the disperse system to transform towards equilibrium. Whereas chemical reactions may accompany the processes or external pressures may support them, the main driving force for sintering is the excess of surface free energy of the disperse system [2] . Theoretical concepts for the early stages of sintering, therefore, concentrate on the contact region between neighbouring particles, where during sintering the initial point-like contact transforms into a sintering neck, replacing a part of the original particle surface by the much smaller neck surface. It is well understood that variations of the surface curvature at particle contacts cause changes in the chemical potential of atoms close to the surface, and the resulting gradients of lattice vacancy concentration are responsible for the directed transport of atoms via volume, grain boundary or surface diffusion. By this concept, the growth of contacts can be theoretically described in good agreement with experimental observations. The annihilation of vacancies at the contact grain boundary explains the shrinkage of the body by the approach of particle centres [4] , [5] , [6] . In real systems, the processes are much more complex even if only one component is present. The complications can arise from geometrical factors (particle shape, particle-size distribution) and from the microstructure (polycrystalline particles, dislocations in the contact region) [2] , [4] , [5] , [6] , [7] , [8] , [9] , [10] . As it is of crucial importance for the understanding of the behaviour of real powder systems, innumerable studies have aimed at such special features of the sintering processes over the past decades. Although sintering models explain the overall behaviour of the multiparticle system on the basis of next-neighbour interactions (two-particle model), it is still an open debate whether entire particles can rearrange into a denser configuration due to the high mobility of atoms at the contact grain boundary [7] , [8] , [9] , [10] . As the diffusion of a small portion of grain boundary atoms would cause the movement of all atoms of the particle, it is common to speak of cooperative transport processes in this context. In general, each particle in the sintering powder in relation to its neighbours could perform a simple translation; it could roll or it could rotate. Here, with 'rotation' we denote the movement of a particle around its own centre, whereas 'rolling' is the revolution of a particle along another particle's perimeter. Rolling is slipless, whereas rotation within a bulk of connected particles involves surface sliding and therefore friction. Obviously, particle-size distributions will result in spatially varying rates of particle-centre approach and a complex particle shape can cause asymmetric necks. Both induce particle motion [7] . A further potential driving force for particle rolling and rotation is the contact grain boundary energy [11] . After initial crystal misorientations at particle contacts have been introduced by the random orientation of each powder particle, the system will tend to reach a state with lower grain boundary energy by adjusting the misorientations [12] , [13] , [14] , [15] . Clear experimental evidence of particle motion during sintering was obtained in previous studies for one-dimensional rows of powder particles and for two-dimensional particle arrays as these situations can be easily observed with traditional methods [16] , [17] , [18] . A quantitative analysis of three-dimensional particle systems is just about to become feasible and is expected to yield a clearly different picture, because other than in 1D or 2D model systems, particle movements in 3D are highly frustrated due to the packing of the particles. High-resolution synchrotron computed tomography (SCT) permits tracking individual particles non-destructively in 3D, provided the appropriate image analysis tools are available. Bernard et al . [19] used ex-situ SCT; Vagnon et al . [20] and Lame et al . [21] , [22] used in-situ SCT to investigate the sintering of glass, copper and steel powders and studied densification, neck size, particle coordination and pore distribution. Nöthe et al . [23] were able to quantify particle sintering in 3D by measuring the changes of the particle-centre positions and of the angles between the lines connecting the centres of neighbouring particles, but the measurement did not allow for a full analysis of the transport process. The aim of the present work was to obtain quantitative evidence of all possible processes, that is, translation, rolling and rotation of powder particles in a 3D packing of loose powder during sintering by first drilling marker holes into the surface of spherical copper particles. A disordered bulk of such particles, containing one or even two holes, was then sintered, while high-resolution and high-speed synchrotron tomography [24] , [25] , [26] were used to measure the rotation angle with respect to a particular particle centre between sinter steps. As monocrystalline and approximately monosized spheres (radii 80−100 μm) were used, the effects of varying rates of centre approach and asymmetric sinter necks were considered negligible and a possible influence of particle-size distribution was minimized. The sintering conditions chosen ensured that the bulk is in early stages of sintering at all times, that is, the particles were still well separated by necks ( Supplementary Fig. S3) . Sintering of free particles and particles inside a confining tube is compared. 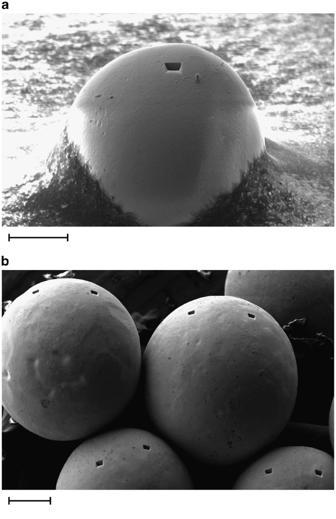Figure 1: Monocrystalline copper spheres used for the sinter experiments. (a) Sphere containing a 5×5×8 μm3marker hole, used for sample I (still embedded in conductive resin here). Scale bar, 20 μm. (b) Particles with two marker holes, each 8×8×12 μm3large, used for sample II. Scale bar, 50 μm. Sintering in a silica capillary Sample I contained 300 particles of the single-hole type shown in Figure 1a , filled into a silica capillary with 1.3 mm inner diameter. The holes are so small that it is unlikely that they are located in the contact area between two particles and influence sintering (see Supplementary Methods) . During tomography, the specimen was heated up continuously at 10 K min −1 in an inert gas atmosphere. Individual tomograms were continuously acquired in situ , which took 85 s for each tomogram. In all, 180 particles were visible in the final tomograms and were used for the analysis (see Supplementary Table S1) . Figure 1: Monocrystalline copper spheres used for the sinter experiments. ( a ) Sphere containing a 5×5×8 μm 3 marker hole, used for sample I (still embedded in conductive resin here). Scale bar, 20 μm. ( b ) Particles with two marker holes, each 8×8×12 μm 3 large, used for sample II. Scale bar, 50 μm. 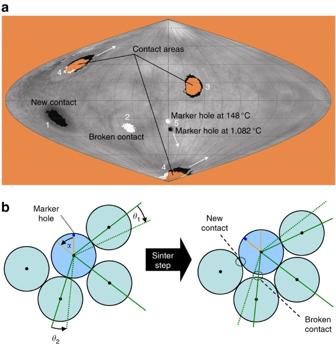Figure 2: Phenomena encountered during sintering. (a) Difference between two sinusoidal projections (also known as Mercator projection, shown here with a 20° grid for both the polar angle from −90° to 90° and the azimuthal angle from −180° to 180°) representing the first (started at 148 °C) and the last (started at 1,082 °C) tomogram of an individual copper sphere containing a marker hole (sample I). White areas are contact areas (2) or marker holes (5) visible in the first but not in the last sintering tomogram. Black areas show contact areas (1) or marker holes (5) visible in the last but not in the first tomogram. Orange colour marks permanent contact areas (3, 4) or areas outside the particle. (b) Sketch of changes around a central particle (given in blue) surrounded by various particles (given in green) as observed during sintering: creation and breakage of interparticle contacts due to particle motion, particle rolling by anglesθ1,θ2and intrinsic rotation by angleα. Full size image The difference between the first and the last tomograms taken of sample I during sintering is given in Figure 2a . An individual copper sphere is displayed as a sinusoidal projection. The data reveal a newly formed interparticle contact (1), a contact that has broken during sintering (2), the growth of a contact that has kept its position (3), two contacts that have moved in the directions marked by white arrows (4) and the marker hole (5) that has moved significantly more than the interparticle contacts and in yet another direction. Figure 2b explains these findings in a schematic way and, in particular, defines the rolling angles θ i of adjacent particles—represented by the displacement of the contact points—and the intrinsic rotation angle α —expressed by the shift of the marker hole. Figure 2: Phenomena encountered during sintering. ( a ) Difference between two sinusoidal projections (also known as Mercator projection, shown here with a 20° grid for both the polar angle from −90° to 90° and the azimuthal angle from −180° to 180°) representing the first (started at 148 °C) and the last (started at 1,082 °C) tomogram of an individual copper sphere containing a marker hole (sample I). White areas are contact areas (2) or marker holes (5) visible in the first but not in the last sintering tomogram. Black areas show contact areas (1) or marker holes (5) visible in the last but not in the first tomogram. Orange colour marks permanent contact areas (3, 4) or areas outside the particle. ( b ) Sketch of changes around a central particle (given in blue) surrounded by various particles (given in green) as observed during sintering: creation and breakage of interparticle contacts due to particle motion, particle rolling by angles θ 1 , θ 2 and intrinsic rotation by angle α . Full size image Rolling and rotation angles The quantitative analysis of particle rolling and rotation movements was carried out using the procedures described in the Methods section. In the following, double-averaged rolling angles are used: the angles θ i are first averaged over all the contacting particles i of a given sphere, after which an average over all such spheres is calculated. The resulting mean rolling angle is therefore a global average for each tomogram. The rotation angle α for each sphere containing a marker is averaged to a mean angle . Angles are always averaged as absolute values without taking into account their direction, however after adjusting the frame of reference (see Supplementary Fig. S7) . Sample I, sintered in the silica capillary, exhibits both particle rolling with respect to the interparticle contacts ( Fig. 3 , broken black line) and intrinsic rotations expressed by the marker rotations ( Fig. 3 , full black line). Both increase continuously throughout sintering. The cumulated average rotation angle at 1,082 °C was about 4°, about twice as high as the corresponding rolling angle . The scatter of the individual rotations is ±3°, more than 3 times the corresponding scatter of the rolling angles. 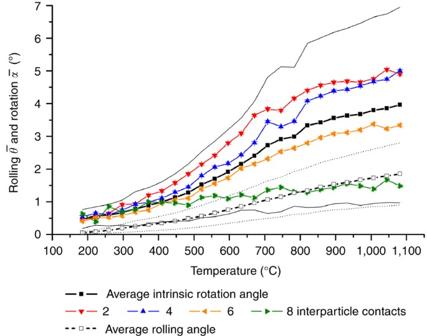Figure 3: Rolling and rotation of copper spheres during sintering in sample I. Globally averaged cumulative particle-rolling angles(black thick broken line) and particle-rotation angles(black thick full line) versus temperature in sample I. The fine black lines show the scatter band of the intrinsic rotations, the fine broken lines denote the scatter band of the rolling angles. The temperatures given refer to the starting point of each sinter step. Coloured symbols refer to a breakdown of the marker rotations with respect to the number of interparticle contacts after the first sinter step. All data are given with respect to the first sinter step (starting at 148 °C). Both scatters are shown as a scatter band in Figure 3 . The magnitude of intrinsic rotation is one of the main results of our study. Note that the angle would have been π /2 times larger if two marker holes had been used (see Supplementary Methods) , bringing it up from 2.1 to 3.3 times the rolling angle. The rotation angle of a given sphere strongly depends on the number of interparticle contacts, as exemplified in Figure 3 , showing a breakdown into contributions for spheres with 2, 4, 6 and 8 contacts. The rotation angles were smaller for spheres that were in contact with more other spheres. This also applies for the scatter of the values (not shown). The initial density at 142 °C was approximately half the theoretical full density and remained largely unchanged during sintering. The average number of contact partners increased from 4.1 to 4.9 during sintering up to 1,082 °C. Figure 3: Rolling and rotation of copper spheres during sintering in sample I. Globally averaged cumulative particle-rolling angles (black thick broken line) and particle-rotation angles (black thick full line) versus temperature in sample I. The fine black lines show the scatter band of the intrinsic rotations, the fine broken lines denote the scatter band of the rolling angles. The temperatures given refer to the starting point of each sinter step. Coloured symbols refer to a breakdown of the marker rotations with respect to the number of interparticle contacts after the first sinter step. All data are given with respect to the first sinter step (starting at 148 °C). Full size image Free sintering of particles For free sintering, sample II, which contained 250 particles of the double-hole type ( Fig. 1b ), was used. The reason for this extra effort was to determine the rotation angles more precisely, because exploratory experiments had shown that without the constraining capillary the rotation and rolling angles were much smaller. Moreover, the two holes in each particle allowed for the unambiguous determination of all particle movements (in the unlikely case that the axis of the rotation coincides with the bisecting line of the angle between the two holes and the sphere centre, a 180° rotation would not be detected. As sample II shows maximum rotation angles of <2°, this special case does not apply). Tomography was carried out ex-situ at room temperature after defined sintering steps at a given temperature: pre-sintering at 650 °C in the capillary, then free sintering at 750, 850, 950 and 1,050 °C for 10 min each, and finally at 1,050 °C for 1 h, all in inert gas. The analysis was based on 170 spheres, but only for 20 spheres the marker pairs could be tracked throughout the sintering stage (see Supplementary Table S1) . 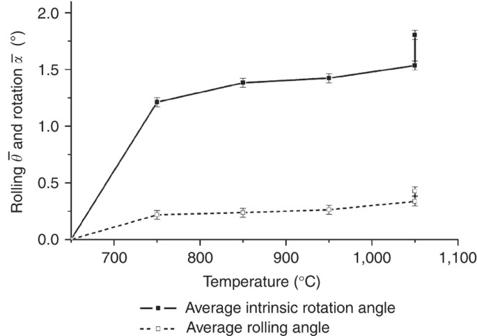Figure 4: Rolling and rotation of copper spheres during sintering in sample II. Anglesandversus temperature for sample II. Values given are with respect to the stage after pre-sintering at 650 °C. The error bars represent the error of the angle measurement, 0.04°. The results for the freely sintered sample II are displayed in Figure 4 . Both angles increase most during the first temperature step after pre-sintering. An initial rotation of 1.2° was followed by a small but continuous increase during isochronal heating, reaching a cumulated angle of 1.5° at 1,050 °C, and a further increase up to 1.8° during 1 h of isothermal holding at that temperature. The rolling angles reached only less than 1/4 of the rotation values. Sample II shows, in comparison with sample I, a smaller increase of the average coordination number from 4.3 to 4.55. Figure 4: Rolling and rotation of copper spheres during sintering in sample II. Angles and versus temperature for sample II. Values given are with respect to the stage after pre-sintering at 650 °C. The error bars represent the error of the angle measurement, 0.04°. Full size image The particle-rolling angle of the individual sphere chosen for display in Figure 2b was θ =2.1° (average over neighbours), whereas the marker rotated by α =8.8° at 1,082 °C (both values are above the averaged angles). This shows that the particles have performed an independent intrinsic rotation despite the restrictions imposed by the contacting neighbour spheres. In the literature, particle rolling is discussed in terms of variants of the two-particle model. Such models only describe rolling motions of particles on top of each other and do not predict the occurrence of intrinsic rotations. For this, the mechanism of contact grain boundary sliding has to be introduced as an additional, simultaneous mechanism. The driving force for the individual particle rotation is assumed to be the minimization of its total grain boundary energy, which is affected by both rolling and rotation. In samples with large, spherical particles of similar size, both inhomogeneous shrinkage due to spatially varying centre approach and asymmetric sinter necks are not expected to occur. The particle network in a 3D sample inhibits rolling significantly because there are no degrees of freedom even if neighbouring particles roll as well, that is, the system is frustrated. Consequentially, the total grain boundary of a particle can only be lowered by intrinsic rotations, and grain boundaries slide with respect to each other. To further elucidate the role of the grain boundary energy in particle rotation, a theoretical model would be required that quantifies grain boundary energy as a function of misorientation and allows to determine this contribution quantitatively. The more the neighbouring particles were connected to a sphere, the lower the intrinsic rotation angle α was (see Fig. 3 ). On the one hand, each interparticle contact contributes to the resistance against rotation, while on the other hand the crystallographic misorientation between a neighbour and the central particle provides the driving force for rotation. Frictional resistance scales linearly with the coordination number N , but the driving force is, on average, sublinear in N because the forces due to the various misorientation angles statistically distributed in 3D increasingly cancel out with higher N as simulations have shown (see Fig. 5 ). Therefore, particles that were bonded to fewer neighbours contributed more to the overall rotation. 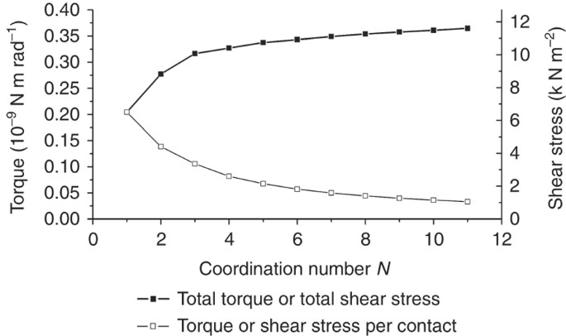Figure 5: Stresses on particles with varying number of neighbours. Torque (or shear stress) exerted on a spherical particle by a shell of neighbours, the crystallographic orientations of which are statistically distributed (seeSupplementary Methods). Values were calculated using real spatial arrangements of a central sphere andNcontact partners, which were extracted from tomograms. Based on a large number of computer-generated random crystallographic orientations of the contact partners with respect to the central particle, the average torque (or shear stress) was calculated. The value normalized byNis also given. No value forN=12 is given because no such configuration was found in the tomograms. Figure 5: Stresses on particles with varying number of neighbours. Torque (or shear stress) exerted on a spherical particle by a shell of neighbours, the crystallographic orientations of which are statistically distributed (see Supplementary Methods ). Values were calculated using real spatial arrangements of a central sphere and N contact partners, which were extracted from tomograms. Based on a large number of computer-generated random crystallographic orientations of the contact partners with respect to the central particle, the average torque (or shear stress) was calculated. The value normalized by N is also given. No value for N =12 is given because no such configuration was found in the tomograms. Full size image The strong influence of using a silica capillary as a particle container is evident from Figures 3 and 4 . Caused by the different thermal expansion coefficients of copper and quartz, the capillary exerted a radial compressional stress on the sample during heating. The particles rearranged with respect to each other to accommodate the effective pressure. In addition, the additional pressure enhanced the sinter activity and by that the diffusion rate. Combined, this leads to the higher rolling and rotation angles observed for sample I compared with sample II. This difference is also reflected in the changes of average coordination number. In sample I, the coordination increased from 4.1 to 4.9, while in sample II it increased from 4.3 to 4.55, that is, the stronger rolling in sample I led to more new contacts between particles. We compare this effect of constrained sintering with the results presented by Lange [27] , who discusses the breakup of contacts in composites and constrained shrinkage. This is practically the inverted constraint found in the silica capillary. A promotion of contact formation and growth is expected and was observed by us. Note that the ratios between rotation and rolling angles for samples I and II get very similar, that is, about 3.3:1 and 4.5:1, if one takes into account the underestimation of α for the spheres containing just one hole (see Supplementary Methods ). In conclusion, particles in early stages of sintering not only roll with respect to their interparticle contacts, but also rotate by much larger angles around their own centres even though they are firmly bonded to neighbouring particles. The crystallographic misorientation energy is strong enough to overcome the resistance between contacting particles and to allow for grain boundary sliding. An external pressure further accelerates this process. The rotations observed in 3D arrangements decrease with a growing number of contacts. The well-known 1D and 2D test arrangements exhibit more extensive rotations than 3D samples. In future work, one could identify the crystallographic orientations of the individual spheres in various sintering stages by including further methods such as electron backscatter diffraction, 3D X-ray contrast tomography [28] , [29] or 3D X-ray diffraction [30] , [31] , [32] , [33] , [34] . Combined with in-situ SCT analysis, one would be able to measure all rotations during the sintering process and to match the respective crystallographic orientations of all particles. Such experimental data should allow one to develop an improved theoretical description of sintering that includes the driving forces and mechanisms of particle translation, rolling and rotation. Computer simulations of particle rearrangements and the calculation of contact grain boundary energies would further contribute to the understanding of details and will help to achieve this goal. A generalized model should also include factors such as local particle arrangement, particle size, size distribution and type and composition of the material. Materials Spherical mono-crystalline copper particles with radii between 80 and 100 μm were produced by reducing CuO, producing Cu droplets, solidifying and then by selecting spherical particles (see Supplementary Fig. S1) . Several hundred particles were marked with either one or two extremely small boreholes each that were drilled using a focused ion beam (see Fig. 1 and Supplementary Methods ). Such marker holes are shown in Figure 1 and Supplementary Figure S2 . Tomography Synchrotron X-ray tomography was carried out either in situ (in the furnace) during sintering at beamline ID15a of the European Synchrotron Radiation Facility or ex-situ between two sinter steps at the BAMLine of the synchrotron BESSY-II. Tomographic reconstruction by filtered backprojection yielded 3D data sets that showed the individual particles and the marker holes as seen in Supplementary Figures S2b and S3a . 3D data analysis The 3D data sets were treated with a software especially developed for the purpose of this study. Analysis took place in three steps: (i) Identification of individual particles in each tomogram: determination of centre positions and radii with an accuracy of 0.1 voxel (volume pixel) ( Supplementary Figs S4 and S5 ), labelling of particles to allow for tracking throughout sintering and identification of marker holes and their positions ( Supplementary Fig. S6 and Supplementary Movies 1 and 2 ). (ii) Analysis of neighbourhoods of each particle: identification of contact partners, calculation of coordination vectors ( Supplementary Movie 3 ). (iii) Analysis of changes between different tomograms, that is, between sinter steps: calculation of rolling and rotation angles ( Supplementary Fig. S7 ) with an accuracy of 0.04° (see Supplementary Methods ). Note that for the complicated geometry in the early stages of sintering, the resolution of the images was not high enough to clearly visualize sinter necks and to determine their radii. How to cite this article: Grupp, R. et al . Cooperative material transport during the early stage of sintering. Nat. Commun. 2:298 doi: 10.1038/ncomms1300 (2011).